Noise-induced quantum coherence drives photo-carrier generation dynamics at polymeric semiconductor heterojunctions Here we report on an exciton/lattice model of the electronic dynamics of primary photo excitations in a polymeric semiconductor heterojunction that includes both polymer π -stacking, energetic disorder and phonon relaxation. Our model indicates that that in polymer/fulerene heterojunction systems, resonant tunnelling processes brought about by environmental fluctuations couple photo excitations directly to photocurrent producing charge-transfer states on <100 fs time scales. Moreover, we find this process to be independent of the location of energetic disorder in the system, and hence we expect exciton fission via resonant tunnelling to polarons to be a ubiquitous feature of these systems. Photovoltaic diodes based on blends of semiconductor polymers and fullerene derivatives now produce power conversion efficiencies exceeding 10% under standard solar illumination [1] . This indicates that photocarriers can be generated efficiently in well-optimized organic heterostructures, but the mechanism for converting highly bound Frenkel excitons to photocarriers is not understood in spite of vigorous, multidisciplinary research activity. A detailed mechanistic understanding of primary charge generation dynamics is of key fundamental importance in the development of organic solar cells, and we propose it to be generally important in photoinduced charge-transfer processes in condensed matter. Recent spectroscopic measurements on organic photovoltaic systems have reported that charged photo excitations can be generated on ≤100-fs time scales [2] , [3] , [4] , [5] , [6] , [7] , [8] , [9] , [10] ; however, full charge separation to produce photocarriers is expected to be energetically expensive given strong Coulombic barriers due to the low dielectric constant in molecular semiconductors. Nonetheless, experiments by Gélinas et al. [11] in which Stark-effect signatures in transient absorption spectra were analysed to probe the local electric field as charge separation proceeds, indicate that electrons and holes separate by ~40 Å over the first 100 fs and evolve further on picosecond time scales to produce unbound charge pairs. Concurrently, Provencher et al. (FP, manuscript in preparation) have demonstrated, via transient resonance Raman measurements, clear polaronic vibrational signatures on sub-100 fs on the polymer backbone, with very limited molecular reorganization or vibrational relaxation following the ultrafast step. Such spectacularly and apparently universally rapid through-space charge-transfer between excitons on the polymer backbone and acceptors across the heterojunction would be difficult to rationalize within Marcus theory using a localized basis without invoking unphysical distance dependence of tunnelling rate constants [12] . Polymer microstructural probes have revealed general relationships between disorder, aggregation and electronic properties in polymeric semiconductors [13] . Moreover, aggregation (ordering) can be perturbed by varying the blend ratio and composition of donor and acceptor polymers [14] . On one hand, energetic disorder at the interface would provide a free energy gradient for localized charge-transfer states to escape to the asymptotic regions. In essence, the localized polarons in the interfacial region could escape into a band of highly mobile polarons away from the heterojunction region [15] . On the other hand, energetic disorder in the regions away from the interface would provide an entropic driving force by increasing the density of localized polaron states away from the interfacial region, allowing the polarons to hop or diffuse away from the interface before recombination could take place [16] . It has also been suggested that in polymer/fullerene blends, interfacial exciton fission is facilitated by charge-delocalization alone the interface, which provide a lower barrier for fission with the excess energy provided by thermally-hot vibronic dynamics [17] . Finally, a report by Bakulin et al. [18] indicates that when relaxed charge-transfer excitons are pushed with an infrared pulse, they increase photocurrent via delocalized states rather than by energy gradient-driven hopping. Upon photo excitation, the system is prepared in an energy eigenstate or superposition of energy eigenstates of the system with precisely defined phase relations—coherences—that evolve in time according to the time-dependent Schrödinger equation. Such coherences can arise from the optical absorption process, or they can be induced by the bath. The noisy bath also induces loss of coherence (decoherence) of such a quantum system by the same fluctuation spectrum that induced coherence, by performing rapid measurements on the system that it prepared. As a result of dephasing or decoherence, the system evolves into a statistical mixture of possible states, which may involve both localized (exciton) and delocalized (charge-separated) eigenstates in organic bulk heterojunction materials. Within the framework of this paper, the outcome of the coherence dynamics does not depend on whether the excitation is impulsive, as in ultrafast spectroscopies, or continuous, as in solar illumination. Indeed, the coherence dynamics that we discuss are unrelated to optical coherence of the excitation source. We report upon rigorous quantum calculations that underscore the role that quantum coherence and energy fluctuations may play in the production of charge-separated states in polymeric type-II heterojunction devices. Our model is based upon a Frenkel exciton lattice model parameterized to describe the π -electronic states of a polymeric semiconductor type-II heterojunction [19] , [20] , [21] , [22] . Similar noise-induced coherent processes may also enhance the quantum efficiency in light–harvesting complexes [23] , [24] , [25] , may be exploited to reduce radiative recombination in photovoltaics cells [26] , [27] , and may be relevant in quantum information applications [28] . The key message of our work is that the noise spectrum associated with the zero-point motion of the molecular lattice vibrations that couple to the electronic optical photoexcitation and that are involved with molecular reorganization on longer time scales, lead to state-to-state off-diagonal couplings that induce transitions between excitons localized on a polymer chain and delocalized charge-separated states in which the hole and the electron are sufficiently far apart across the heterojunction such that charge carriers can be readily produced. Exciton lattice model To explore the role of coherence and noise-induced tunnelling, we constructed a fully quantum mechanical/finite temperature model for a polymer heterojunction consisting of eight parallel stacked polymers each with five sites oriented perpendicular to the heterojunction interface as sketched in Fig. 1 . Details of the model itself are given in the Methods section of this paper. In brief, each site contributes a valance and a conduction-band Wannier orbital and the electronic ground state is where each site is doubly occupied. We estimate the interchain hopping term to be an order of magnitude smaller than the intrachain hopping term, t ⊥ ≈ t ∥ /10, such that electron or hole motion along the chains is easier than hopping between chains. Single electron/hole excitations from the ground state are considered within configuration interaction (CI) theory. Each site also contributes two localized phonon modes that modulate the local energy gap at each site. Linear coupling between localized phonons give rise to optical phonon bands that are delocalized over each polymer chain. 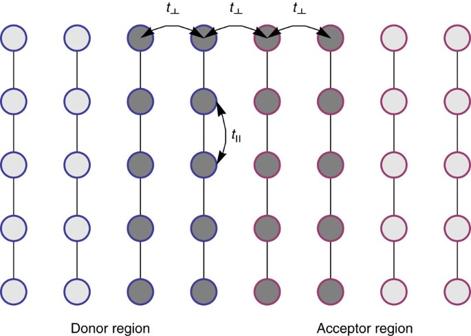Figure 1: Lattice model. The model shows parallel-aligned chains and location of heterojunction boundary. Indicated are the intrachain (t∥) and interchain (t⊥) hopping integrals. Shaded regions correspond to the asymptotic (light grey) or interfacial regions (dark grey). Figure 1: Lattice model. The model shows parallel-aligned chains and location of heterojunction boundary. Indicated are the intrachain ( t ∥ ) and interchain ( t ⊥ ) hopping integrals. Shaded regions correspond to the asymptotic (light grey) or interfacial regions (dark grey). Full size image To gain insight into the role of environmental noise in coupling electronic states, let us consider a model consisting of only two electronic levels separated by an energy difference Δ and coupled to a noisy phonon environment that modulates the local dipole fields and introduces an instantaneous off-diagonal coupling, δV ( t ). In terms of the model above, the two uncoupled states are eigenstates of the dressed Hamiltonian and Δ is the renormalized energy gap, and δV ( t ) is the off-diagonal coupling at a given instant in time. This reduced model follows naturally from the complete model discussed below. State-to-state quantum coherence is induced by the phonon bath via δV ( t ). The dynamics of the coupled system are described by where are the Pauli matrices in a basis of kets |0 and |1 . On average, the off-diagonal coupling =0 and the two states are uncoupled. However, fluctuations about the average given by where S ( ω ) is the spectral density of the coupling to the environment, introduce uncertainty in the energy of the system. 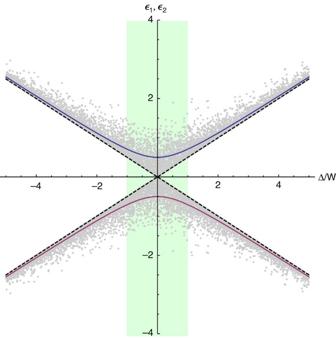Figure 2: Energy eigenvalues distribution equation (1) versus energy gap Δ. The solid curves give the noise averaged eigenvalues and dashed lines are the bare energy levels ±Δ/2. Green shaded region denotes the regime where the off-diagonal noise induces tunnelling between states. Figure 2 shows the energy eigenvalues of equation 1 for multiple samplings of the off-diagonal coupling δV ( t ) with fixed W =1. The superimposed red and blue curves give the average energy eigenvalue at each Δ. These correspond to the eigenvalues Figure 2: Energy eigenvalues distribution equation (1) versus energy gap Δ. The solid curves give the noise averaged eigenvalues and dashed lines are the bare energy levels ±Δ/2. Green shaded region denotes the regime where the off-diagonal noise induces tunnelling between states. Full size image of the noise-averaged Hamiltonian and is the average energy gap. Factoring out a common phase factor, we can write the time-evolved state as where ϕ ( t ) = t is the relative phase for amplitude oscillations between the basis states and a =cos( θ ) is taken as a constant coefficient given by the cosine of the mixing angle, tan2 θ = W /Δ. Fluctuations about the average energy gap lead to an uncertainty in the relative phase between the two states composing the superposition. If we consider the time evolution of a state under the noisy conditions, we can identify two limiting regimes. One is the resonant tunnelling regime where the fluctuations are greater than the gap, W >>Δ and we can make the approximation In this regime, the uncertainty in the phase grows as δ ϕ ( t ) Wt /, and we define a decoherence rate as = W /. Second, when W <<Δ, the coupling is perturbative, and the phase uncertainty grows as δ ϕ ( t ) W 2 t /2Δ, and we define a decoherence rate of = W 2 /2Δ. The role of coherence becomes clear when we consider the population transition rates between states. One can readily write the equations of motion for both the coherences and populations and show that they reduce to that of a damped oscillator with a decay constant given by As T d → 0, the transition rate vanishes. This is the quantum Zeno effect whereby rapid quantum measurements at a rate given by on the system collapses any superposition states that form due to the interactions and suppresses transitions between states. On the other hand, long-lived coherences can facilitate quantum transitions between otherwise weakly coupled states. In the resonant tunnelling regime considered here, where the coupling between states is due to the phonon fluctuations, the fluctuations generate coherences and give rise to damped Rabi oscillations between otherwise uncoupled states. Such coherences may be exploited in the case where an initial photoexcitation (exciton) is in the resonant tunnelling regime with states that are not photoexcited directly, such as nearby charge-transfer states. Such non-thermalized ‘hot exciton’ states have been implicated recently as important precursors in the generation of photocurrent in organic photovoltaics since they undergo fission within the first 50 fs following excitation, creating both interfacial charge-transfer states and polaron species in low bandgap polymer systems [6] , [7] . In essence, as the energy offset between donor and acceptor materials is increased, an increasing density of long-range charge-transfer states (that is, polarons) becomes isoenergetic with the photoexcited excitonic state. Once the energy difference between a charge-separated state and the exciton becomes small compared with their root mean squared coupling, W , resonant tunnelling will occur even if on average the two states are uncoupled on average. Interfacial states To incorporate a heterojunction within our model, we add an energy offset Δ E between chains #4 and #5 such that all site energies to the left and right of the interface are shifted by the offset. At sufficient offset, this provides the necessary driving force such that the lowest lying excitation corresponds to a charge-transfer state pinned to the heterojunction interface. In Fig. 3 we show a representative series of states produced by our model with Δ E =0.5 eV of bias between the donor and acceptor regions. In the states shown here, we have not included the reorganization of the lattice. As such, these states would correspond the vertical excitations from the ground state. With this amount of bias, the lowest lying excitation corresponds to an interfacial charge-transfer state (exciplex) with a positive valence band hole localized on chain #4 and a negative conduction-band electron localized on chain #5. The exciplex is delocalized over the entire length of the chains and corresponds to a bound electron/hole pair undergoing ‘particle in a box’ type motion along the length of the two chains. Within our model, this state is 0.21 eV lower in energy than the excitonic state shown in (b) and carries some oscillator strength due to contributions from excitonic (geminate) electron–hole configurations. State (b) is an excitonic state located in the ‘acceptor’ region. This state consists of geminate electron/hole configurations localized on sites #27–#29 with some contributions coming from nearby chains. This particular state carries the majority of the oscillator strength to the ground state. The state shown in Fig. 3c lies 0.12 eV above the exciton and corresponds to the case where the hole has been transferred from the acceptor phase to the donor phase over a distance corresponding to the stacking distance of three chains. This type of state carries no oscillator strength and can not be directly excited by photo absorption from the ground state. 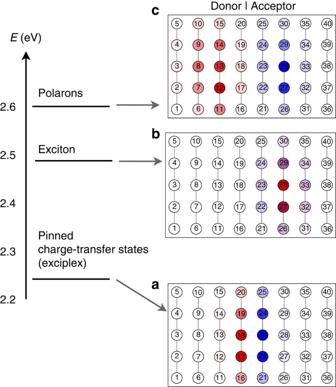Figure 3: Ménagerie of the low-lying interfacial excited states. Red/blue shading on each site corresponds to positive (red) or negative (blue) excess charge. (a) Charge-transfer (exciplex) state that is pinned to the interface (E=2.25 eV). Notice that in going from the exciton state (b) to state (c), the hole has been shifted by three polymer chains. (b) Exciton localized about site #28 in the acceptor phase (E=2.46 eV). (c) Charge-transfer/polaron state. (E=2.58 eV). Figure 3: Ménagerie of the low-lying interfacial excited states. Red/blue shading on each site corresponds to positive (red) or negative (blue) excess charge. ( a ) Charge-transfer (exciplex) state that is pinned to the interface ( E =2.25 eV). Notice that in going from the exciton state (b) to state (c), the hole has been shifted by three polymer chains. ( b ) Exciton localized about site #28 in the acceptor phase ( E =2.46 eV). ( c ) Charge-transfer/polaron state. ( E =2.58 eV). Full size image In the presence of an energy offset at the interface, the lowest energy single excitations are composed of electron/hole configurations pinned along the interface (that is, exciplex states). Even though charge separation has occurred, little or no photocurrent can be produced since the binding energy of the exciplex is greater than the thermal energy. In order to produce current, the electron and hole must overcome their mutual Coulombic attraction and be separated at a distance R >2 e 2 /(3 ∈ k B T ) (assuming a homogeneous 3D medium with dielectric constant ∈ ). Within our model, we define current-producing states as any elementary configuration with the positive hole on the outer most donor chain and the negative electron on the outer most acceptor chain. Such states serve as gateway states for charges to escape from the local heterojunction region [29] . Interfacial disorder To explore the role of interfacial disorder, we include a small amount of gaussian noise ( σ / t ∥ =0.2) in the local HOMO-LUMO gaps in either the region close to the interface or in the regions away from the interface. We shall refer to the two as the ‘ordered-disordered-ordered’ model (ODO) and ‘disordered-ordered-disordered’ model (DOD), respectively. In Fig. 4 we show the average density of states produced by our model as the energy offset between the donor and acceptor region is increased, sampled over 100 realizations of the model. 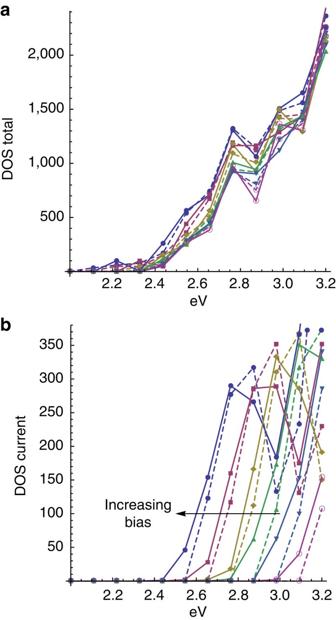Figure 4: Density of states. (a) Density of electronic excited states for both ODO (dashed) and DOD (solid) for increasing interfacial bias. (purple: ΔE=0 to blue: ΔE=0.5eV.) (b) Computed absorption profiles (solid blue and red) and density of current producing states (lines/points) for increasing interfacial bias. Blue absorption peaks correspond to the ΔE=0.5 eV offset cases and the red correspond to the ΔE=0 eV lattice. Both ODO and DOD cases are shown. The curves with data points correspond to the density of current producing states with increasing bias from ΔE=0 to 0.5 eV. Dashed=ODO and solid=DOD. Figure 4: Density of states. ( a ) Density of electronic excited states for both ODO (dashed) and DOD (solid) for increasing interfacial bias. (purple: Δ E =0 to blue: Δ E =0.5 eV .) ( b ) Computed absorption profiles (solid blue and red) and density of current producing states (lines/points) for increasing interfacial bias. Blue absorption peaks correspond to the Δ E =0.5 eV offset cases and the red correspond to the Δ E =0 eV lattice. Both ODO and DOD cases are shown. The curves with data points correspond to the density of current producing states with increasing bias from Δ E =0 to 0.5 eV. Dashed=ODO and solid=DOD. Full size image Figure 4a shows the total density of states produced by both the ODO and DOD models with increasing interfacial bias from Δ E =0 to Δ E =0.5 eV. Increasing the interfacial bias generally produces a shift towards lower energy states composed primarily of charge-transfer states pinned to the donor–acceptor interface. The averaged density of states appears to be insensitive to whether or not the interface is disordered or ordered within the context of our model, although the DOD model does appear to have a higher density of low-lying charge-transfer states than the ODO model. In Fig. 4b , we superimpose the absorption line shapes for both the ODO and DOD models along with the density of ‘current producing’ states as defined by requiring the states to have a threshold density of 10% of their electron/hole configurations on two outermost polymer chains corresponding to states with maximal charge separation. Clearly, increasing the interfacial bias shifts the fraction of states capable of producing current towards lower energies to the extent that they begin to overlap the absorption spectrum of the system. It should also be noted that the energetic onset for producing current is somewhat higher for the DOD cases suggesting that disorder at the interfacial region may facilitate efficient charge separation as suggested by Forrest [15] , [30] . In Fig. 5 , we show energy versus average distance of separation (in units of the lattice constant) between charges for both the ODO (blue points) and DOD (red points) cases for the 0.5 eV biased model. Both cases give interfacial CT states in which the electron and hole are on neighbouring chains separated by the interface and undergo ‘particle in a box’ like motion along the interface. In the ODO case, these states are spread over a wide energy range reflecting the energetic disorder at the interface whereas in the DOD case, the energy spread is very narrow. Once the electron and hole have been separated by three or more chains, the distributions are similar reflecting the fact that at least one of the particles is sampling a random energy landscape. It is important to note that in both cases, the distribution of polaron states with charges separated by two or more chains overlaps the exciton absorption spectrum centred at 2.5 eV. Thus, even small fluctuations in the exciton/phonon coupling will lead to tunnelling transitions from the exciton states to the polaron states. 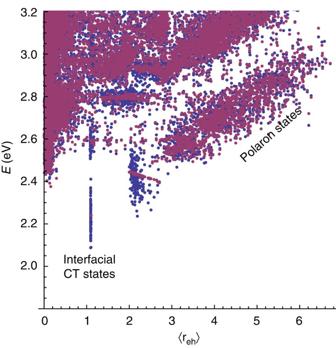Figure 5: Energy versus charge separation distance. The ODO model (blue) and the DOD model (red). Interfacial disorder increases the density of charge-transfer states. Figure 5: Energy versus charge separation distance. The ODO model (blue) and the DOD model (red). Interfacial disorder increases the density of charge-transfer states. Full size image Exciton dissociation rates In Fig. 6a , we show the distribution of noise-averaged interstate couplings between the primary exciton and each of its neighbouring states for the ODO polymer model with a Δ E =0.5 eV offset (sampled over multiple realizations of the lattice). States with E < E ex are predominantly interfacially bound electron–hole pairs (exciplex states). On average, these lower-lying states are coupled very weakly to the primary exciton indicating that relaxation to the lower-lying pinned charge-separated state proceeds via a sequence of microstates. It is surprising, however, that in many cases, the coupling between the exciton to states that are immediately higher in energy are on the order of the energy difference between the primary exciton and the final state. This puts initial (primary exciton) and the polaron states into the strong coupling or resonant tunnelling regime. Since the majority of the states with large couplings correspond to current producing states as defined above, comparing this plot to the density of current producing states one can conclude that the primary exciton can decay directly into the current producing states by resonant tunnelling induced by coupling to the phonon bath. 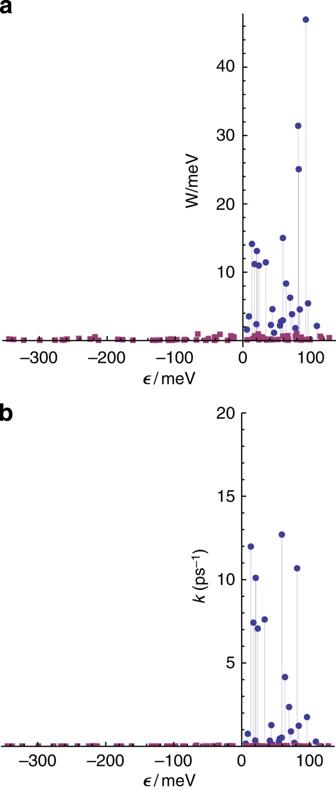Figure 6: Couplings and transition rates. (a) Distribution of couplings and (b) golden rule rates between primary exciton and nearby states at 10 K. Blue points correspond to transition from the primary exciton to polaronic states. Figure 6: Couplings and transition rates. ( a ) Distribution of couplings and ( b ) golden rule rates between primary exciton and nearby states at 10 K. Blue points correspond to transition from the primary exciton to polaronic states. Full size image In Fig. 6b , we show the distribution of golden rule rate constants for transitions originating from the primary exciton (again sampled over multiple realizations of the lattice). defining as the average rate to all nearby higher energy states and as the average rate to all lower energy states, we can estimate the time scale for exciton fission into current producing states as 1/ =35 fs and the time scale for exciton fission into pinned charge-transfer states as 1/ =43 ps. Both of these estimates are consistent with a wide-range of recent experimental evidence indicating that excitons decay into current producing states on time scales of <100 fs. We presented here a lattice model for the interfacial electronic states of a polymer–polymer bulk–heterojunction interface. With increasing band offset, a sizable density of ‘gateway’ states is brought into a resonance with the primary photo excitation. As the energy difference decreases couplings due to phonon fluctuations become equivalent the energy difference between the states, leading to long-range resonant tunnelling of charges away from the initial excitation on an average time scale of 35 fs. Taking the spacing between polymer chains to be ≈4 Å over this time scale, the electron or hole would tunnel ≈12–15 Å away from the site of the initial excitation within 35 fs following excitation. Moreover, given the universal nature of our model, we propose that that direct tunnelling to current producing states assisted by phonon fluctuations plays a ubiquitous role in the ultrafast dissociation of excitons in organic bulk heterojunction cells. While this paper was under review, a related paper was published by Tamura and Burghardt [17] that supports the notion of hot exciton fission assisted by vibronic processes. An important distinction between our work presented here and ref. 17 is that we propose that excitons dissociate directly into quasi-free carrier states rather than via the intermediate interfacial (pinned) CT states. The direct dissociation mechanism suggested by our model is consistent with recent experiments reported in refs 11 discussed in the Introduction of this paper. Heterojuction lattice model In our paper, we employ a two-band exciton/phonon model we described previously modified as to include both stacking and a band offset to define a heterojunction domain [19] , [20] , [21] , [22] , [29] , [31] , [32] . Each site contributes a valance and conduction-band Wannier orbital and the ground state consists of each site being doubly occupied. The important distinction between the present model and that for a single chain is that we estimate the interchain hopping term is an order of magnitude smaller than the intrachain hopping term t ⊥ ≈ t ∥ /10. Thus, electron or hole motion along the chains is easier than hopping between chains. Single electron/hole excitations from the ground state are considered within CI theory that includes all singlet electron/hole configurations. Each local site also contributes two localized phonon modes that modulate the energy gap at each site and give rise to optical phonon bands that are delocalized across each chain. No explicit interchain vibronic coupling was included in our model. The two bands included correspond to the Franck–Condon active modes that contribute to the absorption and fluorescence spectra of conjugated polymer containing phenylene groups such as poly-phenylene-vinylene. Specifically, these correspond to low frequency torsional modes with frequencies and the higher frequency C=C stretching modes that are well known to be coupled to the π -electronic states in poly-phenylene-type conjugated polymer systems. We have used this approach previously to describe the energetics, dynamics and spectroscopy of polymer-based donor–acceptor systems and diodes [19] , [22] , [32] . The model can provide the necessary input for describing the dynamics of a polymer-based photovoltaic cell [33] , [34] , [35] . A similar lattice model for a bulk heterojunction was presented recently by Troisi that includes many of the features of our model, but does not include explicit phonons and electronic transitions between states are introduced via the semiclassical Marcus theory [36] . The energetics and time scales produced by our model are consistent with photon echo experiments on MEH-PPV systems [37] and with the fully atomistic quantum/classical molecular dynamics simulations on phthalocyanine/fullerene interfaces reported in ref. 6 . With the exception as noted above, the electronic couplings and electron/phonon couplings used here are the same as reported in our earlier works on exciton dissociation at interfaces. [34] , [35] , [38] A complete listing of the interaction terms and parameters is given in ref. 20 . A copy of our exciton code is also available on SourceForge.com or upon request. Within the context of a CI calculation, our state space is constructed by considering singlet electron/hole excitations of the form where removed an electron with spin σ from an occupied valance orbital (or HOMO) on site m (creating a hole) and places it in the unfilled conduction orbital (or LUMO) of site n . The vacuum state |0 is where each valance orbital is doubly occupied. We consider the electronic states and transitions between excitonic and polaronic states in a system of stacked polymer chains using a Hamitonian of the general form: [19] , [20] , [21] , [22] . The electronic part reflects the CI of single excitations for a generic two-band polymer in a localized basis. The configurations | m = taken over valence and conduction-band Wannier functions and | m represent geminate ( = m ) and charge-transfer ( ≠ m ) e-h pairs. is parameterized from the π -band structure of extended PPV. Since the conjugated backbone is alternant, one-body CI integrals F mn = of the band structure operator obey electron hole symmetry with =− t r . The important distinction between the present model and that for a single chain is that we estimate the interchain hopping term is an order of magnitude smaller than the intrachain hopping term t ⊥ ≈ t ∥ /10. The electron–hole interactions are spin dependent with In this work, we only consider singlet excitations; however, the model can be employed for triplets. Assuming zero-differential overlap except for geminate orbitals, we take into account only true Coulomb and exchange terms With the exception of geminate Wannier functions, orbital overlap is small such that the two-body interactions are limited to Coulomb and exchange integrals reflecting e–h attraction and spin-exchange coupling non-geminate configurations with r =| m − n | and r o a characteristic length for each interaction. We also include transition dipole–dipole integrals coupling only geminate singlet electron–hole pairs, The electron–phonon coupling term assumes that the localized conduction/valence levels ± ∈ o and nearest-neighbor transfer integrals ± t 1 are modulated by linear coupling to the phonons. Correspondingly, the phonon term consists of two sets of interacting local oscillators, giving rise to two dispersed optical phonon branches centred at 1600 and 100 cm −1 , respectively. These frequencies correspond to the C=C bond stretches and ring torsions in PPV both of which dominate the Franck-Condon activity of the lowest optical transitions. Thus, by empirical adjustment of electron–phonon coupling strength in , we can compute accurate absorption and emission band shapes for PPV chains, reflecting conjugation-length dependence, vibronic structure and Stokes shifts. [20] Diagonalizing and yields vertical excited states with energies and normal modes with frequencies ω ξ , which allow us to transform the electron–phonon coupling term within the diabatic representation. With the exception of the energy offsets and interchain hopping terms, a complete listing of the electron/hole interaction terms and parameters is given in ref. 20 . Inclusion of phonon bath Taking the electronic ground state of the system as a reference and assuming that the electronic states are coupled linearly to a common set of phonon modes, we arrive a generic form for the Hamiltonian: where are electronic states with energies , and [ a q , ] = δ qq ′ are the creation/annihilation operators for phonons with frequency { ω q }. The electronic and and phonon degrees of freedom are coupled via diagonal and off-diagonal terms, g ijq . This form is particularly useful for our purposes since we can compute the energies and couplings either with quantum chemical methods or the exciton model we describe later in this report. Central to our model is the notion that off-diagonal couplings are due fluctuations in the phonon degrees of freedom drive transitions between electronic states. To compute these, we break equation 14 into diagonal and off-diagonal terms and perform a polaron transform using the unitary transformation [33] , [39] , [40] under which our transformed Hamiltonian can be written in terms of the diagonal elements where the renormalized electronic energies are and off-diagonal terms Under this unitary transformation, the diagonal parts of the electron/phonon Hamiltonian become with renormalized electronic energies Applying the polaron transformation to the off-diagonal terms gives the renormalized couplings as At this point, it is useful to connect the various terms in the phonon dressed Hamiltonian with specific physical parameters. The terms involving ( g nnj − g mmj )/ ω j are related to the reorganized energy difference between the two states. where S j is the Huang-Rhys factor for phonon mode j . This is related to the Franck–Condon factor describing the overlap between the v j =1 vibronic state in one electronic state with the v j =0 vibronic state in the other. Likewise, the energy difference between the renormalized energy gaps is related to the driving force of the state-to-state transition, In the transformed picture, the electronic transitions from state | n to | m are dressed by the excitations of all the normal phonon modes. Transforming to the interaction representation and performing a trace over the phonons gives the spectral density in terms of the autocorrelation of the electron/phonon coupling operators. Integrating over phonon frequency gives the root mean squared energy fluctuations and the average coupling strength between each pair of states. Finally, the Fermi golden rule transition rates can be computed by evaluating S nm ( ) at the transition frequency, . The derivation and explicit form for these in terms of the non-adiabatic electron/phonon couplings is quite lengthy and is given in ref. 33 . How to cite this article : Bittner, E. R. and Silva, C. Noise-induced quantum coherence drives photo-carrier generation dynamics at polymeric semiconductor heterojunctions. Nat. Commun. 5:3119 doi: 10.1038/ncomms4119 (2014).